Non-redundant requirement for CXCR3 signalling during tumoricidal T-cell trafficking across tumour vascular checkpoints T-cell trafficking at vascular sites has emerged as a key step in antitumour immunity. Chemokines are credited with guiding the multistep recruitment of CD8 + T cells across tumour vessels. However, the multiplicity of chemokines within tumours has obscured the contributions of individual chemokine receptor/chemokine pairs to this process. Moreover, recent studies have challenged whether T cells require chemokine receptor signalling at effector sites. Here we investigate the hierarchy of chemokine receptor requirements during T-cell trafficking to murine and human melanoma. These studies reveal a non-redundant role for G αi -coupled CXCR3 in stabilizing intravascular adhesion and extravasation of adoptively transferred CD8 + effectors that is indispensable for therapeutic efficacy. In contrast, functional CCR2 and CCR5 on CD8 + effectors fail to support trafficking despite the presence of intratumoral cognate chemokines. Taken together, these studies identify CXCR3-mediated trafficking at the tumour vascular interface as a critical checkpoint to effective T-cell-based cancer immunotherapy. The immune contexture is widely recognized as an important determinant of overall survival in cancer patients [1] . In particular, the presence of cytotoxic CD8 + T cells at high density within tumour tissue is beneficial in multiple cancer types including colorectal, ovarian and melanoma, and can be a better prognostic indicator of patient outcome than traditional tumour-node-metastasis (TNM) staging [1] , [2] , [3] , [4] , [5] , [6] . Active areas of research seek to improve T-cell-mediated immunity in patients by focusing on therapeutics that manipulate either the T-cell arm of antitumour immunity or the tumour microenvironment where T cells execute their effector functions [7] , [8] , [9] . The frequency of tumour-specific T cells and their cytotoxic function can be boosted through dendritic cell (DC) vaccination, adoptive T-cell transfer (ACT) therapy, or administration of checkpoint blockade inhibitors (for example, targeting immunosuppressive molecules such as cytotoxic T-lymphocyte-associated protein 4 or programmed-death-1/programmed-death ligand 1 (PD-L1)) and has led to durable responses in a subset of patients [8] , [10] , [11] , [12] , [13] . Alternatively, we and others have converted the tumour microenvironment from relatively ‘low’ to ‘high’ sites of T-cell infiltration in preclinical studies using Toll-like receptor (TLR) agonists, interferons (IFNs), antagonists of endothelin B and angiogenic factors, or interleukin-6 (IL-6)-dependent strategies [9] , [14] , [15] , [16] , [17] . Fundamental to the efficacy of all T-cell-based immunotherapy is the requirement for blood-borne T cells to gain entry across tumour vascular gateways, to engage in contact-dependent lysis of neoplastic targets. Given the importance of intratumoral localization of T cells for antitumour immunity, there is surprisingly little known about the trafficking cues necessary to direct extravasation of effector T cells across tumour vessels. Chemokines are considered strong candidates for this process based on their well-established role in T-cell trafficking to lymphoid organs [18] . In lymph nodes, for example, the interaction between G αi -protein-coupled chemokine receptors (for example, CCR7) on naive T cells and chemokine (CCL21) displayed on the lumenal surface of blood vessels is an obligate step for triggering LFA-1-dependent stable adhesion and subsequent transendothelial migration [18] , [19] . Insight into the role of chemokines in the tumour microenvironment stems from correlative studies linking T-cell accumulation with multiple chemokine receptors on effector T cells and/or chemokines within the tumour locale [1] , [20] , [21] . In this regard, expression of CXCR3 on circulating T cells or its chemokine ligands, CXCL9 and CXCL10, in tumour tissues is associated with elevated intratumoral T-cell infiltration and a favourable outcome in melanoma and colorectal cancer patients [1] , [20] , [21] , [22] . Similar clinical evidence connects CCR5 and its ligands (CCL3, CCL4 and CCL5), as well as CCR2 and its ligand CCL2, to intratumoral T-cell infiltration and disease-free survival [1] , [20] , [21] . These observations are suggestive of redundant functions by chemokine receptors during T-cell homing into tumours, although chemokines could alternatively orchestrate T-cell activities within the tumour interstitium (for example, proliferation, survival, retention or egress) [19] . Moreover, the prototypical role for chemokines has recently been challenged by reports in non-tumorigenic inflammatory settings that CD8 + effector T cells with high LFA-1 expression bypass chemokine requirements for stable adhesion within vessels [23] , [24] . Thus, in the absence of a head-to-head comparison of the chemokine receptor usage at the tumour vascular interface, it remains unclear whether chemokines are operative during T-cell entry into tumours or if there is any preferential role for individual chemokine receptors/chemokine pairs during extravasation. Here we investigated the hierarchy of chemokine receptor requirements during T-cell trafficking by tracking the fate of adoptively transferred CD8 + effector T cells in murine and human melanoma tumours. We compared the functions of three chemokine receptors previously implicated in intratumoral CD8 + effector T-cell infiltration (that is, CXCR3, CCR5 and CCR2) in tumours expressing complementary chemokine ligands. These studies unexpectedly reveal a non-redundant requirement for the CXCR3-CXCL9/CXCL10 axis for CD8 + T-cell trafficking within the intravascular space that could not be predicted from static profiling of intratumoral chemokines or their receptors on T cells. We further establish a causal link between CXCR3-dependent trafficking and the efficacy of ACT therapy. These findings identify CXCR3 interactions with cognate chemokines within the vessel wall as a critical checkpoint dictating the efficacy of T-cell-based cancer immunotherapy. Tumour microenvironment enriched for T-cell chemoattractants To address the chemokine receptor requirements during T-cell homing, we first characterized the chemokine milieu in highly aggressive, orthotopic B16 murine melanoma expressing the surrogate tumour antigen ovalbumin (OVA) [14] . For these studies, we focused on inflammatory chemokines previously implicated in T-cell infiltration in patient tumours [1] , [3] , [9] , [20] . High concentrations ( ∼ 1 ng per mg total protein) of CXCL9, CXCL10 (that is, the two CXCR3 ligands expressed in the C57BL/6 strain [25] ), CCL5 (CCR5 ligand) and CCL2 (CCR2 ligand) were detected in B16-OVA tumour extracts compared with non-inflamed normal skin following subcutaneous (s.c.) injection of phosphate buffered saline (PBS) ( Fig. 1a ). 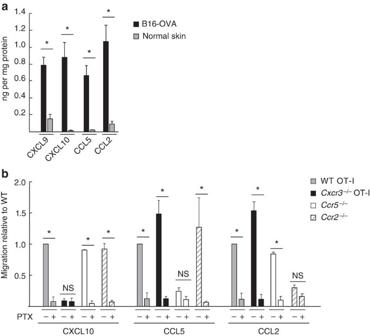Figure 1: Murine CD8+effector T cells express an array of functional chemokine receptors complementary for chemokine ligands present in the tumour microenvironment. (a) Cognate chemokine ligands for CXCR3, CCR5 and CCR2 (that is, CXCL9/CXCL10, CCL5 and CCL2, respectively) were quantified by ELISA in B16-OVA tumour extracts (tumour volume∼400–500 mm3) or in normal skin from tumour-free mice. Data (mean±s.e.m.) are from ≥3 independent experiments (n≥2 mice per group). (b) Transwell assays were performed where fluorescently labelled WT OT-I T cells were admixed with equivalent numbers of chemokine receptor-deficient effector cells and tested for migration to the indicated recombinant chemokines. WT and chemokine receptor-deficient cells were also pretreated with the global G-protein inhibitor PTX and migration was quantified by flow cytometry. Background migration (absence of chemokine) was subtracted from all values. Data (mean±s.e.m.) are represented as migration relative to WT and are from ≥3 independent experiments. (a,b) *P<0.05; NS, not significant; unpaired two-tailed Student’st-test. Figure 1: Murine CD8 + effector T cells express an array of functional chemokine receptors complementary for chemokine ligands present in the tumour microenvironment. ( a ) Cognate chemokine ligands for CXCR3, CCR5 and CCR2 (that is, CXCL9/CXCL10, CCL5 and CCL2, respectively) were quantified by ELISA in B16-OVA tumour extracts (tumour volume ∼ 400–500 mm 3 ) or in normal skin from tumour-free mice. Data (mean±s.e.m.) are from ≥3 independent experiments ( n ≥2 mice per group). ( b ) Transwell assays were performed where fluorescently labelled WT OT-I T cells were admixed with equivalent numbers of chemokine receptor-deficient effector cells and tested for migration to the indicated recombinant chemokines. WT and chemokine receptor-deficient cells were also pretreated with the global G-protein inhibitor PTX and migration was quantified by flow cytometry. Background migration (absence of chemokine) was subtracted from all values. Data (mean±s.e.m.) are represented as migration relative to WT and are from ≥3 independent experiments. ( a , b ) * P <0.05; NS, not significant; unpaired two-tailed Student’s t -test. Full size image Complementary studies profiled CD8 + effector T cells for functional receptors specific for the inflammatory chemokines found in the tumour microenvironment. Chemotactic activity was tested in vitro for CD8 + T cells from OVA-specific OT-I transgenic mice (wild-type (WT)) or chemokine receptor-deficient mice that were activated ex vivo , to simulate the expansion of T cells for clinical ACT immunotherapy [12] , [14] , [26] . WT OT-I effector populations (>96% CD8 + CD44 hi , Supplementary Fig. 1a ) exhibited strong migration to recombinant CXCL9, CXCL10, CCL5 and CCL2, which was blocked by pertussis toxin (PTX), a global inhibitor of G αi protein-coupled chemokine receptor signalling ( Fig. 1b ). Genetic deletion of Cxcr3 (crossed on an OT-I background; Cxcr3 −/− OT-I) or Ccr5 and Ccr2 (on a C57BL/6 background) was further shown to specifically block T-cell migration to its cognate ligands without impairing the response to other ligands ( Fig. 1b ). CD8 + CD44 hi T cells activated ex vivo exhibited a CXCR3 hi CCR2 int/lo CCR5 int/lo phenotype, which was also typical of CD8 + T cells activated in vivo (that is, detected in draining nodes following DC vaccination or tumour implantation; Supplementary Fig. 1b ). Collectively, these data indicate that CD8 + effector T cells express a repertoire of functional chemokine receptors, which would be expected to guide trafficking to chemokine-rich tumours in situ . CXCR3 signalling obligate for intratumoral T-cell trafficking Short-term (1 h) competitive homing assays were used [14] , [27] to determine whether G αi -chemokine signalling was obligatory for T-cell trafficking in B16-OVA. In these assays, WT effector OT-I cells were admixed at a 1:1 ratio with PTX-pretreated WT OT-I T cells (labelled with different tracking dyes) before intravenous (i.v.) ACT ( Fig. 2a ). After 1 h, the ratio of T cells was determined in tumour tissues by flow cytometry and data are reported for homing relative to untreated WT OT-I cells. This 1-h time-frame enabled us to discriminate chemokine functions specifically at the vessel wall, as it is sufficient for cells to complete the steps leading to extravasation [14] , but not long enough for other processes to occur that influence the extent of T-cell infiltration (that is, proliferation in situ , survival, retention and egress). Homing of PTX-treated OT-I was less efficient than WT OT-I, as indicated by the 1:3 ratio of PTX:WT cells recovered in tumours ( Fig. 2b ). This was in contrast to control experiments where a 1:1 ratio of intratumoral WT:WT cells was detected. Access of effector T cells to the spleen via the peripheral circulation was not affected by functional chemokine receptor status ( Fig. 2b ). These data establish that G αi -coupled chemokine receptor signalling is necessary for effector CD8 + T cell homing in tumours. 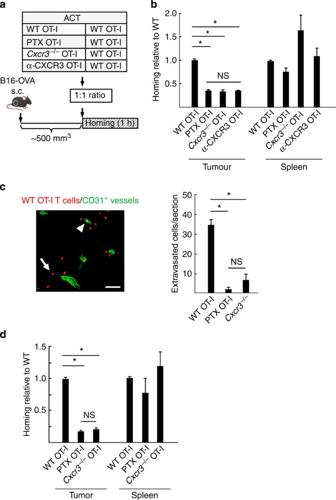Figure 2: CXCR3 is obligatory for murine CD8+effector T-cell trafficking to melanomain vivo. (a) Experimental scheme for short-term (1 h) competitive homing studies. The groups used for ACT included WT OT-I cells co-mixed at a 1:1 ratio with WT OT-I cells, WT OT-I cells pretreated with PTX,Cxcr3−/−OT-I cells or WT OT-I cells pretreated with α-CXCR3-blocking Ab. Fluorescent-labelled CD8+effector T cells were injected i.v. into mice with established B16-OVA tumours (tumour volume∼400–500 mm3) and homing was evaluated after 1 h. (b) Data represent ratio of adoptively transferred T cells relative to WT determined by flow cytometry in tumours and spleens following competitive homing assays. (c) The number of WT (red) orCxcr3−/−cells, which successfully extravasated into underlying interstitium was quantified in histological tumour sections counterstained with CD31-specific Ab (green) to demark vessels. A representative photomicrograph of homed WT OT-I cells is shown with an example of an extravasated cell indicated by a white arrow and a vessel-associated cell noted by a white arrowhead. Scale bar, 100 μm. (d) Ratio of adoptively transferred T cells recovered in B16-OVA tumour-bearing mice pretreated with STT (39.5±0.5 °C for 6 h). PTX, pertussis toxin; α-CXCR3, CXCR3-blocking Ab. (b–d) All data (mean±s.e.m.) are from ≥3 independent experiments (n≥2 mice per group). *P<0.001; NS, not significant; unpaired two-tailed Student’st-test. Figure 2: CXCR3 is obligatory for murine CD8 + effector T-cell trafficking to melanoma in vivo . ( a ) Experimental scheme for short-term (1 h) competitive homing studies. The groups used for ACT included WT OT-I cells co-mixed at a 1:1 ratio with WT OT-I cells, WT OT-I cells pretreated with PTX, Cxcr3 −/− OT-I cells or WT OT-I cells pretreated with α-CXCR3-blocking Ab. Fluorescent-labelled CD8 + effector T cells were injected i.v. into mice with established B16-OVA tumours (tumour volume ∼ 400–500 mm 3 ) and homing was evaluated after 1 h. ( b ) Data represent ratio of adoptively transferred T cells relative to WT determined by flow cytometry in tumours and spleens following competitive homing assays. ( c ) The number of WT (red) or Cxcr3 −/− cells, which successfully extravasated into underlying interstitium was quantified in histological tumour sections counterstained with CD31-specific Ab (green) to demark vessels. A representative photomicrograph of homed WT OT-I cells is shown with an example of an extravasated cell indicated by a white arrow and a vessel-associated cell noted by a white arrowhead. Scale bar, 100 μm. ( d ) Ratio of adoptively transferred T cells recovered in B16-OVA tumour-bearing mice pretreated with STT (39.5±0.5 °C for 6 h). PTX, pertussis toxin; α-CXCR3, CXCR3-blocking Ab. ( b–d ) All data (mean±s.e.m.) are from ≥3 independent experiments ( n ≥2 mice per group). * P <0.001; NS, not significant; unpaired two-tailed Student’s t -test. Full size image We next investigated whether there was a hierarchy of chemokine receptor usage during extravasation into tumour tissue. Initial studies focused on CXCR3 requirements for the entry of adoptively transferred effector T cells in competitive (1 h) homing assays in which WT OT-I cells were admixed with Cxcr3 −/− OT-I T cells or with OT-I cells pre-treated with a CXCR3-blocking antibody (Ab). Surprisingly, despite expression of functional CCR5 and CCR2 ( Fig. 1b ), loss of the single chemokine receptor, CXCR3, reduced T-cell trafficking to the same extent as global blockade of chemokine signalling by PTX ( Fig. 2b ). Further head-to-head comparison of admixed PTX-pretreated and Cxcr3 −/− OT-I cells in the same recipient mice substantiated that CXCR3 accounted for all G αi -coupled chemokine receptor-dependent trafficking by CD8 + effectors in B16-OVA melanoma ( Supplementary Fig. 2a ). Microscopic quantification of homed cells within the interstitium (that is, T cells located outside CD31 + vessels in tumour sections) further demonstrated an absolute requirement for CXCR3 during T-cell extravasation ( Fig. 2c ). Contributions of other chemokine receptors failed to emerge even when the overall rate of trafficking was improved ( ∼ 2-fold) using an IL-6-dependent thermal preconditioning strategy (core body temperature elevated to 39.5±0.5 °C, 6 h) that targets the tumour vasculature to be more permissive for T-cell homing [14] ( Fig. 2d and Supplementary Fig. 2b ). CXCR3 dependence was also evident during endogenous CD8 + T-cell infiltration in tumours implanted in WT mice and Cxcr3 -deficient mice ( Supplementary Fig. 2c ), suggesting that the same CXCR3 bias exists whether T cells are activated ex vivo or in vivo . Collectively, these data establish a non-redundant role for CXCR3-mediated G αi protein signalling during emigration of blood-borne CD8 + effector T cells in the tumour microenvironment. CXCR3 ligands mediate T-cell firm arrest in tumour vessels Our findings demonstrated that CXCR3 is required at some point during the multistep migration process leading to CD8 + effector T-cell migration. These observations prompted our use of epifluorescence intravital microscopy to examine whether CXCR3 plays a prototypical role in triggering T-cell adhesion [18] , [19] within the intravascular space in tumour tissues. As our prior studies established that the frequency of baseline adhesive interactions between effector T cell and tumour vessels is near the lower limit of detection by live imaging [14] , we administered thermal therapy to augment homing in order to interrogate subtle chemokine requirements. PTX uncoupling of G αi protein signalling or genetic deletion of Cxcr3 had no impact on the ability of OT-I cells to initiate rolling interactions within tumour vessels but strongly inhibited the transition to firm arrest ( Fig. 3a ). Notably, WT and Cxcr3 −/− effector OT-I expressed comparable levels of adhesion molecules necessary for rolling and firm arrest (that is, E/P-selectin ligands and CD11a (the α-subunit of LFA-1), respectively; Supplementary Fig. 3a ). The dependence on G αi protein signalling further was not unique to tumour vessels, as PTX-pretreated OT-I effectors exhibited significantly reduced firm arrest of CD8 + effectors in inflamed skin vessels of non-tumour-bearing mice stimulated with the TLR4 agonist, lipopolysaccharide (LPS) ( Supplementary Fig. 3b ). 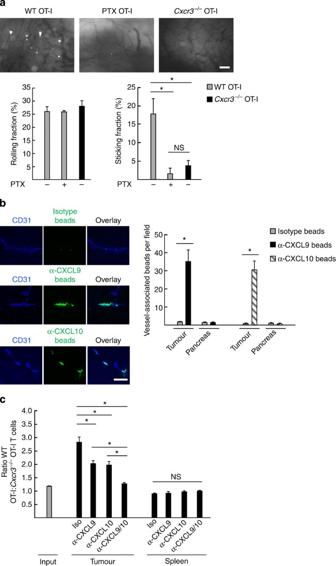Figure 3: Intravascular CXCR3 ligands support stable adhesion of murine CD8+T cells within tumour vesselsin vivo. (a) Representative photomicrographs of intravital microscopy depicting stable interactions of fluorescently tagged WT OT-I cells, WT OT-I cells pretreated with PTX orCxcr3−/−OT-I effector cells within B16-OVA tumour vessels in mice pretreated with STT (core temperature elevated to 39.5±0.5 °C for 6 h). Data (mean±s.e.m.) for rolling fractions and sticking fractions are from ≥3 independent experiments (n≥2 mice per group). *P<0.05. (b) Isotype- and α-CXCL10- or α-CXCL9 Ab-conjugated fluorescent beads (green) were injected into B16-OVA mice by tail vein. Tumour and pancreatic sections were counterstained with anti-CD31 Ab (blue), to identify beads associated with vascular structures. Representative images from tumours containing isotype, α-CXCL9- or α-CXCL10 Ab-conjugated beads are shown. Data (mean±s.e.m.) are of ten fields analysed from paired mice and are from three independent experiments. *P<0.001. (a,b) Scale bars, 100 μm. (c) Mice were treated i.p. with chemokine-neutralizing Ab 3 h before competitive homing assays using WT OT-I andCxcr3−/−OT-I effector T cells. The ratio of WT OT-I:Cxcr3−/−OT-I cells at the time of transfer (input) or within tumour and spleen post-transfer was quantified by flow cytometry. Data (mean±s.e.m.) are from three independent experiments (n=2 mice per group). *P<0.04, compared with isotype or dual Ab treatment. (a–c) Data were analysed by unpaired two-tailed Student’st-test; NS, not significant. Figure 3: Intravascular CXCR3 ligands support stable adhesion of murine CD8 + T cells within tumour vessels in vivo . ( a ) Representative photomicrographs of intravital microscopy depicting stable interactions of fluorescently tagged WT OT-I cells, WT OT-I cells pretreated with PTX or Cxcr3 −/− OT-I effector cells within B16-OVA tumour vessels in mice pretreated with STT (core temperature elevated to 39.5±0.5 °C for 6 h). Data (mean±s.e.m.) for rolling fractions and sticking fractions are from ≥3 independent experiments ( n ≥2 mice per group). * P <0.05. ( b ) Isotype- and α-CXCL10- or α-CXCL9 Ab-conjugated fluorescent beads (green) were injected into B16-OVA mice by tail vein. Tumour and pancreatic sections were counterstained with anti-CD31 Ab (blue), to identify beads associated with vascular structures. Representative images from tumours containing isotype, α-CXCL9- or α-CXCL10 Ab-conjugated beads are shown. Data (mean±s.e.m.) are of ten fields analysed from paired mice and are from three independent experiments. * P <0.001. ( a , b ) Scale bars, 100 μm. ( c ) Mice were treated i.p. with chemokine-neutralizing Ab 3 h before competitive homing assays using WT OT-I and Cxcr3 −/− OT-I effector T cells. The ratio of WT OT-I: Cxcr3 −/− OT-I cells at the time of transfer (input) or within tumour and spleen post-transfer was quantified by flow cytometry. Data (mean±s.e.m.) are from three independent experiments ( n =2 mice per group). * P <0.04, compared with isotype or dual Ab treatment. ( a–c ) Data were analysed by unpaired two-tailed Student’s t -test; NS, not significant. Full size image To determine whether there was a preferential contribution for individual CXCR3 ligands for trafficking, we adapted an approach described previously to visualize membrane-anchored adhesion molecules in lymph node vasculature [28] , to determine which CXCR3 ligands were available in the intravascular space. In the present study, intravascular chemokines were quantified microscopically in tissue sections following i.v. injection of fluorescent beads conjugated with CXCR3 ligand-specific Ab. These studies focused on CXCL9 and CXCL10, as C57BL/6 mice do not express CXCL11 (refs 25 , 29 ). Both CXCL9 and CXCL10 were displayed within tumour vessel walls as indicated by specific accumulation of α-CXCL10 and α-CXCL9 Ab-conjugated beads in CD31 + vessels compared with isotype controls ( Fig. 3b ), whereas CXCR3 ligand-conjugated beads were not evident in normal tissues (for example, pancreas). We then employed a chemokine-blocking strategy in which tumour-bearing mice were pre-treated with blocking Ab to CXCL9, CXCL10 or combined CXCL9/CXCL10 (refs 25 , 30 ) before adoptive transfer of admixed WT: Cxcr3 −/− T cells ( Fig. 3c ). Partial inhibition of CD8 + T-cell homing was observed with single chemokine blockade, whereas complete inhibition occurred on dual targeting of CXCL9 and CXCL10 (that is, as indicated by 1:1 ratio of WT: Cxcr3 −/− cells recovered at tumour sites following dual Ab blockade, which was equivalent to the input ratio; Fig. 3c ). There was no change in the spleen, confirming that the inhibitory effects on intratumoral homing cannot be attributed to Ab-mediated T-cell clearance. Taken together, these data identify CXCR3 interactions with intravascular ligands as a critical step leading to stable adhesion and subsequent transendothelial migration of adoptively transferred CD8 + effector T cells at tumour sites. CCR5 and CCR2 are dispensable for T-cell homing to tumours Results that CCR5 and CCR2 were unable to compensate for loss of CXCR3 in vivo do not exclude the possibility that these chemokine receptors cooperate with CXCR3 to control adhesion in tumour vessels. There is already precedent for cooperativity involving these chemokine receptors [31] , [32] . For example, physical interactions between CCR5 and CXCR4 are required for CXCR4-mediated enhancement of T-cell activation in vitro [32] , whereas simultaneous exposure of cells to CCL2 and CCL5 lowers the threshold for downstream calcium mobilization [31] . To assess whether CCR5 or CCR2 were operative in the context of CXCR3-dependent T-cell trafficking, we first established that CCL5 and CCL2 were also available in the tumour intravascular space, as would be necessary to coordinate with CXCR3 ligands during extravasation ( Fig. 4a ). We then performed competitive homing studies to examine the ability of Cxcr3 −/− , Ccr5 −/− , or Ccr2 −/− CD8 + effector CD8 + T cells to traffic compared with WT ( Fig. 4b ). In these experiments, the T cells used to track homing were from normal C57BL/6 mice, not the OT-I background. Consistent with our results for OT-I cells, trafficking was markedly inhibited by PTX treatment of WT cells or Cxcr3 deficiency, indicating that recognition of cognate tumour-associated antigen is not necessary for CXCR3-dependent T-cell extravasation at tumour loci. Conversely, loss of Ccr2 or Ccr5 did not compromise T-cell entry into B16-OVA tumours or in peripheral sites such as the spleen ( Fig. 4b ). Of note, although CCR2 did not contribute to T-cell trafficking, there was sufficient ligand available to support CCR2-dependent intratumoral recruitment of CD115 + inflammatory monocytes [33] that have high CCR2 expression relative to CD8 + effectors ( Fig. 4c,d and Supplementary Fig. 4 ). As CCL2 and CCL5 have been implicated in T-cell diapedesis in vitro [23] , we also considered whether Ccr5 −/− and Ccr2 −/− T cells were defective in their ability to migrate through tumour vessel walls, which would not be discernible by flow cytometric analysis. Microscopic analysis did not reveal a disproportionate accumulation of adoptively transferred Ccr5 −/− or Ccr2 −/− T cells within tumour vessels nor a concomitant defect in extravasation ( Fig. 4e ). Overall, these data demonstrate that CCR5 and CCR2 are not required to cooperate with CXCR3 during T-cell extravasation across tumour vessels. 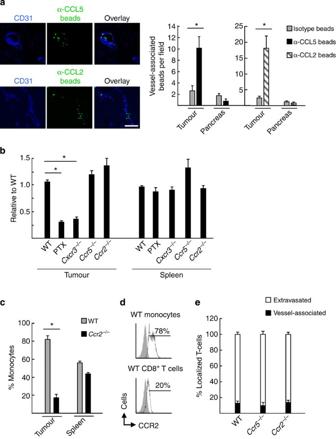Figure 4: Functional cooperativity of CCR5 and CCR2 is not necessary for CXCR3-dependent trafficking of murine CD8+effector T cells to tumours. (a) Isotype- and α-CCL5 or α-CCL2 Ab-conjugated fluorescent beads (green) were injected into B16-OVA mice by tail vein. Tumour and pancreatic sections were counterstained with anti-CD31 Ab (blue), to identify beads associated with vascular structures. Data (mean±s.e.m.) are of ten fields analysed from paired mice from ≥3 independent experiments. *P<0.003. Scale bar, 100 μm. (b) WT effector T cells were comixed at a 1:1 ratio with WT cells, WT cells pretreated with PTX,Cxcr3−/−cells,Ccr5−/−cells orCcr2−/−cells (allex vivoactivated cells>88% CD8+; generated from population of pooled spleen/lymph nodes of mice on C57BL/6 background). Ratio of adoptively transferred T cells relative to WT in tumours or spleens of B16-OVA tumour-bearing mice following short-term competitive homing assays is shown. Data (mean±s.e.m.) are from three independent experiments (n≥2 mice per group). *P<0.001 compared with WT. (c) Per cent of adoptively transferred WT andCcr2−/−inflammatory CD115+monocytes in tumours and spleens of B16-OVA tumour-bearing mice following competitive homing assays. Data (mean±s.e.m.) are from three independent experiments (n=2 mice per group). *P<0.003 compared with WT. (d) Flow cytometric analysis of WT CD8+effector T cells and inflammatory CD115+monocytes for surface expression of CCR2 (unfilled histograms); grey-filled histograms represent isotype control Ab staining. (e) Histological analysis was performed following short-term competitive homing assays between fluorescently labelled WT effector CD8+T cells andCcr5−/−orCcr2−/−effector T cells. The proportion of homed cells, which were vessel-associated or extravasated outside CD31+vessels, are shown. Data (mean±s.e.m.) are from two independent experiments (n=2 mice per group). (a–c,e) Data were analysed by unpaired two-tailed Student’st-test. Figure 4: Functional cooperativity of CCR5 and CCR2 is not necessary for CXCR3-dependent trafficking of murine CD8 + effector T cells to tumours. ( a ) Isotype- and α-CCL5 or α-CCL2 Ab-conjugated fluorescent beads (green) were injected into B16-OVA mice by tail vein. Tumour and pancreatic sections were counterstained with anti-CD31 Ab (blue), to identify beads associated with vascular structures. Data (mean±s.e.m.) are of ten fields analysed from paired mice from ≥3 independent experiments. * P <0.003. Scale bar, 100 μm. ( b ) WT effector T cells were comixed at a 1:1 ratio with WT cells, WT cells pretreated with PTX, Cxcr3 −/− cells, Ccr5 −/− cells or Ccr2 −/− cells (all ex vivo activated cells>88% CD8 + ; generated from population of pooled spleen/lymph nodes of mice on C57BL/6 background). Ratio of adoptively transferred T cells relative to WT in tumours or spleens of B16-OVA tumour-bearing mice following short-term competitive homing assays is shown. Data (mean±s.e.m.) are from three independent experiments ( n ≥2 mice per group). * P <0.001 compared with WT. ( c ) Per cent of adoptively transferred WT and Ccr2 −/− inflammatory CD115 + monocytes in tumours and spleens of B16-OVA tumour-bearing mice following competitive homing assays. Data (mean±s.e.m.) are from three independent experiments ( n =2 mice per group). * P <0.003 compared with WT. ( d ) Flow cytometric analysis of WT CD8 + effector T cells and inflammatory CD115 + monocytes for surface expression of CCR2 (unfilled histograms); grey-filled histograms represent isotype control Ab staining. ( e ) Histological analysis was performed following short-term competitive homing assays between fluorescently labelled WT effector CD8 + T cells and Ccr5 −/− or Ccr2 −/− effector T cells. The proportion of homed cells, which were vessel-associated or extravasated outside CD31 + vessels, are shown. Data (mean±s.e.m.) are from two independent experiments ( n =2 mice per group). ( a – c , e ) Data were analysed by unpaired two-tailed Student’s t -test. Full size image Efficacy of adoptive transfer cell therapy depends on CXCR3 Evidence that CXCR3 directs homing of adoptively transferred CD8 + T cells at the tumour vascular interface prompted us to investigate the relationship between CXCR3 and antitumour immunity. In these studies, we initially characterized the cytotoxic activity of WT and Cxcr3 −/− OT-I T cells in assays where effectors have ready access to cognate targets. Activated Cxcr3 −/− and WT OT-I cells were indistinguishable with respect to IFN-γ and granzyme B expression ( Supplementary Fig. 5a ), and exhibited equivalent specific cytotoxicity against cognate targets in vitro including splenocytes pulsed with SIINFEKL OVA peptide, B16-OVA or OVA-expressing EG7 lymphoma ( Supplementary Fig. 5b-d ). Parallel results were obtained during in vivo cytotoxicity assays against SIINFEKL-pulsed splenocyte targets within the splenic compartment ( Fig. 5a ). These findings are in line with evidence that CXCR3 deficiency does not compromise localization of adoptively transferred CD8 + T cells within the spleen ( Fig. 2b ). 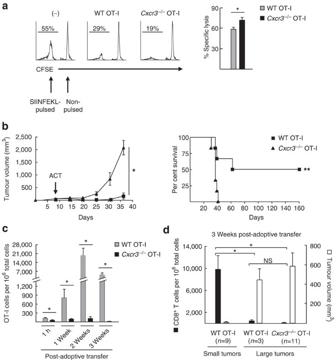Figure 5: Antitumour efficacy of adoptively transferred CD8+effector T cells depends on CXCR3 activity. (a)In vivocytotoxicity of SIINFEKL-pulsed splenocytes in the absence (-) or presence of WT orCxcr3−/−OT-I effector T cells. T cells were transferred into host animals before injection of fluorescently labelled SIINFEKL-pulsed and non-pulsed targets. Spleens were analysed for target cells by flow cytometry after 24 h. Left, representative flow plots of the spleens. Right, per cent specific lysis of SIINFEKL-pulsed targets. Data (mean±s.e.m.) are from two independent experiments (n=2 mice per group). *P<0.05. (b) WT orCxcr3−/−OT-I effector T cells were adoptively transferred into mice bearing B16-OVA tumours; time of administration of ACT therapy is denoted by the arrow. Tumour growth (left) and survival (right) were monitored over time; complete tumour rejection was detected in 50% of mice treated with WT OT-I cells. Data (mean±s.e.m.) are representative of four independent experiments. *P<0.001; **P<0.02; statistical significance of tumour growth, two-way analysis of variance for repeated measures; survival, Kaplan–Meier log rank tests. (c,d) The extent of CD8+CD44+OT-I infiltration and (d) tumour volume were examined at various times after adoptive transfer using tracking dye; *P<0.05; NS, not significant. (b–d)n≥6 mice/group. (a,c,d) Data were analysed by unpaired two-tailed Student’st-test. Figure 5: Antitumour efficacy of adoptively transferred CD8 + effector T cells depends on CXCR3 activity. ( a ) In vivo cytotoxicity of SIINFEKL-pulsed splenocytes in the absence (-) or presence of WT or Cxcr3 −/− OT-I effector T cells. T cells were transferred into host animals before injection of fluorescently labelled SIINFEKL-pulsed and non-pulsed targets. Spleens were analysed for target cells by flow cytometry after 24 h. Left, representative flow plots of the spleens. Right, per cent specific lysis of SIINFEKL-pulsed targets. Data (mean±s.e.m.) are from two independent experiments ( n =2 mice per group). * P <0.05. ( b ) WT or Cxcr3 −/− OT-I effector T cells were adoptively transferred into mice bearing B16-OVA tumours; time of administration of ACT therapy is denoted by the arrow. Tumour growth (left) and survival (right) were monitored over time; complete tumour rejection was detected in 50% of mice treated with WT OT-I cells. Data (mean±s.e.m.) are representative of four independent experiments. * P <0.001; ** P <0.02; statistical significance of tumour growth, two-way analysis of variance for repeated measures; survival, Kaplan–Meier log rank tests. ( c , d ) The extent of CD8 + CD44 + OT-I infiltration and ( d ) tumour volume were examined at various times after adoptive transfer using tracking dye; * P <0.05; NS, not significant. ( b–d ) n ≥6 mice/group. ( a , c , d ) Data were analysed by unpaired two-tailed Student’s t -test. Full size image To test the cytotoxic activity of T cells in tumours where entry depends on CXCR3, we adoptively transferred a single dose of WT or Cxcr3 −/− OT-I effector T cells i.v. into mice and monitored B16-OVA tumour progression. These studies exploited the OT-I T cell receptor (TcR) transgenic model system, to dissect the therapeutic impact of chemokine-dependent trafficking without masking chemokine contributions due to weak TcR affinity/avidity for tumour antigen. WT OT-I T cells caused a significant delay in tumour growth and prolonged survival, with cures detected in some experiments ( Fig. 5b and Supplementary Fig. 6a ). Conversely, CD8 + effectors lacking Cxcr3 provided no therapeutic benefit, compared with untreated controls, in this stringent model where 100% of transferred cells were tumour (OVA) reactive ( Supplementary Fig. 6a ). Kinetic studies performed after adoptive transfer showed a progressive increase in the extent of intratumoral infiltration by WT OT-I cells, but not Cxcr3 −/− OT-I (monitored using tracking dye or CD45 congenic mismatch), underscoring the CXCR3 requirements for tumour immunity ( Fig. 5c and Supplementary Fig. 6b ). In addition, we found that a high intratumoral density of WT OT-I ( ∼ 10,000 OT-I per 10 6 total cells within tumours) correlated directly with tumour control in the majority of mice analysed at 3 weeks post adoptive transfer (that is, tumours <20 mm 3 in 9/12 mice; Fig. 5d ). Conversely, WT OT-I were present at a low density ( ∼ 50 OT-I/10 6 total cells in tumours) in the subgroup of mice in which tumours were progressing (tumours >450 mm 3 in 3/12 mice). Notably, the tumour volume and density of WT OT-I cells detected in progressing tumours was indistinguishable from observations in 100% of mice treated with Cxcr3 −/− OT-I that failed to reject tumours ( Fig. 5d ). These results are consistent with a prior report showing that OT-I must exceed a critical threshold within B16-OVA tumours for ACT immunotherapy to be successful [34] . Collectively, these data indicate that CXCR3-dependent signalling at the tumour vascular barrier is a critical checkpoint for the efficacy of adoptively transferred T cells. Human effector T cells require CXCR3 for homing in melanoma In light of the importance of CXCR3-dependent trafficking for antitumour immunity following ACT therapy in mice, we extended our analysis of chemokine requirements to the trafficking of human effector T cells to human melanoma xenografts comprising the M537 and M888 patient-derived melanoma cell lines [20] , [35] , [36] . We initially profiled chemokine receptor expression by human T cells that were activated and expanded ex vivo using clinical ACT protocols for cancer patients [12] , [26] , [37] . Activated peripheral blood-derived mononuclear cells from normal donors ( n =7) were predominantly CD3 + (>97%) with robust CXCR3 expression on CD8 + cells (that is, the major T-cell subset), whereas CCR2 and CCR5 were highly variable among individual donors as reported previously [20] , [37] , [38] ( Fig. 6a and Supplementary Fig. 7a ). Chemotaxis assays in vitro further validated that activated human T cells expressed functional CXCR3, CCR5 and CCR2, which responded to both human and murine chemokines ( Supplementary Fig. 7b ). As our studies with murine CD8 + effector T cells raised the possibility that limited CCR2 or CCR5 expression might be responsible for the failure to detect CCR2- or CCR5-dependent trafficking to murine melanoma, we selected representative donor T-cell populations for adoptive transfer experiments that dually expressed high CXCR3/CCR2 (donor 1) or high CXCR3/CCR5 (donor 2; Fig. 6a ). 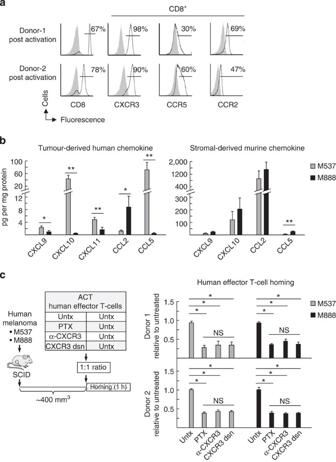Figure 6: Non-redundant requirement for CXCR3 during human effector T-cell trafficking in human melanoma xenografts. (a) Chemokine receptor profile on CD8+T cells (activatedex vivo) from peripheral blood leukocytes of two normal human donors. Grey-filled histograms represent isotype control Ab staining. (b) Concentration of human and murine chemokines in tumour extracts from two human melanoma xenografts (M537 and M888) was determined by Luminex and ELISA, respectively. Data (mean±s.e.m.) are from four independent experiments (n≥4 mice per group) for human chemokines and from ≥2 independent experiments (n≥3 mice per group) for murine chemokines. *P<0.05; **P<0.006, M537 versus M888 tumours. (c) Left, schematic for short-term (1 h) competitive homing studies. The groups used for ACT included untreated (Untx) human effector T cells from donor 1 or donor 2 that were co-mixed at a 1:1 ratio with untreated cells, PTX-pretreated cells, α-CXCR3 Ab-pretreated cells, or cells where CXCR3 was desensitized by exposure to recombinant CXCL10 before transfer into mice (CXCR3 dsn). Right, ratio of adoptively transferred T cells relative to untreated cells in tumours of M537 or M888 tumour-bearing SCID mice following short-term competitive homing assays is shown. PTX, pertussis toxin; α-CXCR3, CXCR3-blocking Ab. Data (mean±s.e.m.) are from ≥2 independent experiments (n=2 mice per group). *P<0.02; NS, not significant. (b,c) Data were analysed by unpaired two-tailed Student’st-test. Figure 6: Non-redundant requirement for CXCR3 during human effector T-cell trafficking in human melanoma xenografts. ( a ) Chemokine receptor profile on CD8 + T cells (activated ex vivo ) from peripheral blood leukocytes of two normal human donors. Grey-filled histograms represent isotype control Ab staining. ( b ) Concentration of human and murine chemokines in tumour extracts from two human melanoma xenografts (M537 and M888) was determined by Luminex and ELISA, respectively. Data (mean±s.e.m.) are from four independent experiments ( n ≥4 mice per group) for human chemokines and from ≥2 independent experiments ( n ≥3 mice per group) for murine chemokines. * P <0.05; ** P <0.006, M537 versus M888 tumours. ( c ) Left, schematic for short-term (1 h) competitive homing studies. The groups used for ACT included untreated (Untx) human effector T cells from donor 1 or donor 2 that were co-mixed at a 1:1 ratio with untreated cells, PTX-pretreated cells, α-CXCR3 Ab-pretreated cells, or cells where CXCR3 was desensitized by exposure to recombinant CXCL10 before transfer into mice (CXCR3 dsn). Right, ratio of adoptively transferred T cells relative to untreated cells in tumours of M537 or M888 tumour-bearing SCID mice following short-term competitive homing assays is shown. PTX, pertussis toxin; α-CXCR3, CXCR3-blocking Ab. Data (mean±s.e.m.) are from ≥2 independent experiments ( n =2 mice per group). * P <0.02; NS, not significant. ( b , c ) Data were analysed by unpaired two-tailed Student’s t -test. Full size image To survey the chemokine milieu available to adoptively transferred T cells in human melanoma xenografts, we measured both tumour-derived (human) and stromal-derived (murine) chemokines produced in the local tumour milieu. Differential production of tumour-derived (human) CXCL9, CXCL10, CXCL11, CCL2 and CCL5 was observed in M537 and M888 xenografts in vivo ( Fig. 6b ), which is largely in line with previous in vitro observations [20] . However, stromal-derived murine chemokines represented the vast majority of local chemokine and were detected at similar levels in M537 and M888 tumour extracts ( Fig. 6b ). Thus, M537 and M888 tumours had similar chemokine microenvironments when considering the combined contributions from both mouse and human chemokines, allowing for chemokine-dependent trafficking to be investigated in both tumour systems. Short-term competitive homing assays were then used to examine CXCR3 contributions during human T-cell trafficking to melanoma xenografts ( Fig. 6c ). CXCR3 activity was specifically disrupted on activated T cells before adoptive transfer with a blocking Ab that reportedly inhibits CXCR3-mediated migration in vitro [39] . As a second method, we desensitized T cells with recombinant CXCL10 to downregulate surface expression of CXCR3 (ref. 40 ). CXCR3 inactivation by these approaches was confirmed by flow cytometry or in vitro chemotaxis assays ( Supplementary Fig. 7c ). Data in Fig. 6c demonstrate that loss of CXCR3 activity by Ab blockade or desensitization diminished homing of T cells from both donor 1 and donor 2 in M537 and M888 melanoma xenografts to the same extent as PTX pretreatment but did not alter localization in the spleen ( Fig. 6c and Supplementary Fig. 8 ). Homed cell populations in tumours were ≥65% CD8 + T cells, which were reflective of the predominantly CD8 + T-cell input population ( Fig. 6a ). Thus, high expression of CCR2 or CCR5 by human effector T cells could not compensate for the absence of CXCR3. The CXCR3 requirement for trafficking in M537 and M888 was further validated in competitive homing assays using murine WT and Cxcr3 −/− CD8 + effector T cells ( Supplementary Fig. 9a,b ). Taken together, these data unequivocally show a non-redundant role for CXCR3 in trafficking of CD8 + human effector T cells in melanoma during ACT immunotherapy. Successful delivery of blood-borne CD8 + effector T cells across the tumour vasculature is recognized as a key determinant of antitumour immunity. However, to date, there is no information about the hierarchy of chemokine receptors that guide tumoricidal T cells into the tumour microenvironment. Here we report on the non-redundant function of CXCR3 and its complementary intravascular ligands during CD8 + T-cell trafficking to tumour tissues. The requirement for CXCR3 is shared by both murine and human CD8 + effector T cells and is necessary for the efficacy of ACT therapy in the B16-OVA tumour model. These findings provide mechanistic insight for observations in cancer patients that CXCR3 expression by circulating T cells and intratumoral CXCR3 ligands are independent indicators of a favourable prognosis [21] , [22] . Surprisingly, CCR5 and CCR2 did not contribute to T-cell trafficking across tumour vessels, despite the presence of cognate chemokines in the tumour microenvironment. These findings highlight the disconnect between functional readouts from in vitro chemotaxis assays and in vivo trafficking. Our results corroborate observations that the chemotactic response to soluble chemokine does not necessarily reflect the pro-adhesive signals delivered by immobilized chemokine on two-dimensional endothelial surfaces [41] , [42] , [43] . Collectively, these studies reveal a unique role for CXCR3/CXCR3 ligands in cancer immunotherapy in vivo that could not be predicted from genomic and proteomic profiling of the inflammatory signature in the tumour microenvironment. Our findings, together with recent reports [23] , [24] , suggest that the dependence of effector T cells on G αi protein signalling at the vascular interface is dictated by the inflammatory context, thus having broad implications outside the tumour milieu. Central to these studies was the discrimination of G αi -dependent trafficking mechanisms using PTX, which irreversibly uncouples G αi protein signalling from chemokine receptor/ligand binding [19] . Our data establish the requirement for PTX-dependent signalling during the transition of CD8 + effector cells from rolling to firm arrest in tumour vessels as well as in normal vessels in the context of LPS-induced systemic inflammation. This requirement is in line with evidence that CXCR3 contributes to CD8 + T-cell localization in inflamed normal skin [19] , [44] , [45] as well as the prevailing view whereby chemokines trigger a conformational change in LFA-1, resulting in an ∼ 500-fold increased affinity for ICAM-1 that stabilizes intravascular adhesion [19] , [46] . Intermediate chemokine receptor requirements were described during delayed-type hypersensitivity responses in which CD8 + effectors bypass G αi protein signalling during the firm adhesion step and instead rely primarily on CCR2 during transendothelial migration [23] . Cardiac allograft rejection models represent the other end of the spectrum where extravasation of CD8 + effector T cells is completely independent of G αi protein signalling [24] . The reasons for these differential chemokine requirements are unclear, but probably involve variability within the tissue microenvironment rather than T-cell behavior, as each of these disparate reports used activated OT-I CD8 + effector T cells. One possibility is that differences in downstream TLR signalling following induction of local delayed-type hypersensitivity by injection of complete freund’s adjuvant [23] (via TLR2 (ref. 47 )) or by systemic LPS administration (via TLR4 (ref. 48 )) account for distinct chemokine receptor requirements in the intravascular space [49] . A key difference between the allograft model and our studies is that G αi -independent trafficking occurs as a consequence of TcR activation by transplant antigens presented by vascular endothelium or nearby DCs [24] . In contrast, results of the current study combined with our previous findings [14] indicate that trafficking of murine T cells or normal donor-derived human CD8 + effectors to tumours or inflamed tissues is not antigen restricted, which may serve to reinforce T-cell dependence on intravascular chemokines. Observations that CCR2 and CCR5 do not participate during CD8 + effector T-cell trafficking into melanoma tumours raise questions about how CCR2 supports monocyte homing in the same intravascular chemokine environment. This could be explained, in part, by the recently discovered posttranslational nitration of CCL2, which supports monocyte but not effector T-cell chemotaxis in vitro [38] . Nitrated CCL2 is found in the tumour microenvironment of murine and human colon and pancreatic tumours [38] , presumably modified by nitric oxygen species derived from local protumorigenic myeloid cells. Furthermore, global blockade of peroxynitrite enhances T-cell infiltration and decreases detectable nitrated CCL2 in murine tumours, although a cause-and-effect relationship for these observations remains to be established [38] . The commercial Ab used to detect intravascular CCL2 in our studies does not appear to recognize nitrated CCL2 in tumour tissues [38] (Dr Barbara Molon, personal communication); hence, there may still be a substantial pool of nitrated CCL2 on the intravascular surface, which could preferentially support monocyte trafficking. Differential migratory responses of monocytes and T cells to nitrated CCL2 in vitro have been attributed to higher CCR2 surface expression on monocytes [38] , a distinction that we also observed for murine CD115 + inflammatory monocytes and CD8 + effectors. Evidence that human CD8 + effector T cells expressing high levels of CCR2 or CCR5 failed to use these receptors during trafficking to human melanoma tumours suggests that deficient receptor expression cannot fully account for the selective dependence of CD8 + effectors on CXCR3 in vivo . These results indicate that there may be cell-intrinsic properties that impact chemokine receptor activity in vivo , such as variations in the availability of molecules, which regulate G αi protein signalling downstream of receptor activation. Strong candidates for cell-specific negative regulation include G protein-coupled receptor kinases (GRKs), which phosphorylate the carboxy-terminal intracellular loop of chemokine receptors to prevent the association of heterotrimeric G αβγ complexes [50] , [51] , and regulators of G protein signalling (RGS), which accelerate the exchange of GTP on active G α subunits to limit signal duration [50] , [51] , [52] . Notably, the G protein-coupled receptor kinase-2 (GRK-2) isoform is elevated in activated human T cells compared with monocytes [53] , [54] and is implicated in repressing both CCR2 and CCR5 signalling [55] , [56] . Similarly, elevated expression of regulators of G protein signalling-1 (RGS-1) has been reported in activated T cells compared with peritoneal macrophages [57] . Thus, it is likely that the net balance of regulatory molecules for G αi signalling within cells has a substantial impact on the ability of CD8 + effectors to respond to intravascular CCR2 and CCR5 ligands in tumours. Our data support a scenario whereby CXCR3-dependent delivery of blood-borne T cells at the vascular juncture is a critical step in therapeutic antitumour immunity. As CXCR3, CCR5 and CCR2 are all associated with overall levels of T-cell infiltration and positive outcomes in cancer patients [1] , [20] , [21] , it is tempting to speculate that signalling through these or other G αi -linked receptors support the antitumour activity of CD8 + T cells within the interstitium via mechanisms independent of extravasation. For example, in vitro studies have shown that CXCR3 and CCR5 enhance T-cell activation and proliferation [58] , [59] , whereas CCL2 can increase the cytotoxicity of T cells engineered to co-express CCR2 and chimeric antigen receptors [60] . In addition, ligand engagement of the G αi -coupled leukotriene B4 receptor has been linked to increased accumulation of CD8 + T cells and T-cell-mediated antitumour immunity in a murine cervical cancer model [61] . Although not addressed in the current study, CXCR3 on T cells could also function outside tumour tissues by regulating antitumour immunity within lymphoid organs. In this regard, CXCR3 has already been implicated in non-tumour systems in guiding CD4 + or CD8 + T-cell positioning near antigen-loaded DCs within lymph nodes and the spleen during T-cell priming and the generation of effector populations [25] , [62] . These observations are highly relevant to preclinical and clinical ACT therapy in which the efficacy depends on direct cytotoxic functions of effector T cells within tumours as well as seeding of lymphoid organs by memory T cells, to perpetuate long-term antitumour immunity [8] , [12] , [14] , [18] . In summary, this report identifies the interface between CXCR3 on effector T cells and chemokine ligands within tumour vessels as a critical checkpoint dictating the efficacy of T-cell-based cancer immunotherapy. The experimental strategy used here to interrogate the homing properties of large numbers of transferred T cells is analogous to clinical adoptive transfer protocols where the goal is to massively expand the tumour-specific T-cell pool. As an example, recent studies have shown that it is technically feasible to transfer >120 billion tumour-reactive T cells in a patient in a bolus injection [63] . Given our observations that CXCR3 is also required for intratumoral localization of endogenous CD8 + T cells, it is likely to be that conclusions regarding biased CXCR3 usage are also relevant to other immunotherapies in which a lower frequency of tumour-reactive T cells might be generated. Similar CXCR3 requirements for homing of CD8 + effectors may also be operative in other orthotopic murine tumours such as the PyMT breast tumour model, which exhibits more aggressive growth after implantation in Cxcr3 −/− hosts because of M2 macrophage polarization [64] . These observations provide guidance for which chemokine receptor/chemokine pair could be exploited clinically to improve antitumour immunity. Our results, together with other published studies, demonstrate that there is universally high CXCR3 expression on ex vivo activated human T cells either from normal donors or cancer patients [20] , [37] . Thus, inadequate expression of CXCR3 does not appear to be an obstacle to adoptive T-cell immunotherapy. In contrast, the tumour microenvironment is highly variable with respect to CXCR3 ligand expression [1] , [20] , [21] , [37] . This raises the possibility of using therapeutic strategies to boost CXCR3 ligands in the tumour locale, which could be shuttled out onto the endothelial surface through the process of transcytosis [65] , [66] . Several approaches being studied clinically to promote an antitumorigenic inflammatory gene signature such as administration of TLR ligands (for example, CpG or poly I:C) or IFN-α have been shown in preclinical studies to induce production of CXCR3 ligands by intratumoral stromal cells (fibroblasts, monocytes or CD45 + leukocytes) [9] , [15] , [67] . Commonly used chemotherapeutic agents such as cisplatin and temozolomide similarly boost tumour cell expression of CXCR3 ligands in preclinical melanoma models, paralleling the increases in CXCL9 and CXCL10 gene expression detected in melanoma patient tumours after treatment with dacarbazine [68] . Moreover, intratumoral injection of recombinant CXCL10 or adenovirus encoding CXCL10 reportedly contributes to CD8 + T-cell infiltration and tumour rejection in murine tumours [69] , [70] . Based on our current findings, we would predict that chemokine-targeting strategies further offers promise in an adjuvant setting with ACT therapy, cancer vaccines or checkpoint blockade inhibitors that rescue CD8 + T-cell function by disrupting cytotoxic T-lymphocyte-associated protein 4 and programmed-death-1/PD-L1-mediated immune-suppressive networks [8] , [10] , [11] , [13] . It is noteworthy, in this regard, that elevated CXCL9 expression in patient melanoma specimens correlates with response to PD-L1 blockade therapy [13] . Animals Female, age-matched C57BL/6 and OT-I mice on a CD45.1 background (B6.129S7-Rag1tm1Mom Tg[TcraTcrb]1,100Mjb) (8–12 weeks) were from the National Cancer Institute or Taconic; C57BL/6 with CD45.2 phenotype (B6.SJL-Ptprca Pepcb/BoyJ), C cr5 −/− (B6.129P2-Ccr5tm1Kuz/J) and Ccr2 −/− mice ( B6.129S4-Ccr2tm1Ifc/J) were from Jackson Laboratory and bred in-house along with C xcr3 −/− OT-I (on a C57BL/6/CD45.1 background as described [29] ) and SCID mice (SCID C.B Igh-1b Icr Tac Prkdc scid) in the Roswell Park Department of Laboratory Animal Resources. Animal protocols were approved by the Roswell Park Cancer Institute Institutional Animal Care and Use Committee. Tumour models B16-OVA cells and parental B16 were cultured in complete media (RPMI 1,640 supplemented with 10% FCS, 2 mM L -glutamine, 100 U ml −1 penicillin, 50 μg ml −1 streptomycin and 50 μM β-mercaptoethanol (Invitrogen)). M537 and M888 cells were cultured in complete media lacking β-mercaptoethanol [20] , [35] , [36] . EL4 and EG7 cells were cultured in complete media supplemented with 1 mM sodium pyruvate, MEM non-essential amino acids, 25 mM HEPES (Invitrogen); media for EG7 cells contained 40 μg ml −1 G418 sulfate (Life Technologies). Tumour cells (10 6 ) were injected s.c. in the flank of C57BL/6 mice or SCID mice as previously described [14] , [20] and were used for experimental analysis when tumour volume reached ∼ 400–500 mm 3 ( ∼ 10–14 days or 6–8 weeks post implantation for murine and human melanoma, respectively), unless otherwise indicated. T-cell activation ex vivo or in vivo Pooled murine splenocyte/lymph node populations (2 × 10 6 cells per ml) were activated for 2 days in 24-well plates (Corning) coated with anti-mouse CD3 Ab (2.5 μg ml −1 ; catalogue number 550275, clone 145-2C11; BD Biosciences) in complete media (including MEM non-essential amino acids, 20 mM HEPES, 1.5 mM sodium pyruvate), then diluted to 2 × 10 5 cells per ml and expanded for 3 days with recombinant human IL-2 (12.5 ng ml −1 ; Peprotech). Human peripheral blood-derived mononuclear cells were isolated from anonymous normal donor buffy-coats obtained from the Roswell Park blood donor centre by centrifugation on a Ficoll–Hypaque gradient, washed with Hank’s balanced salt solution and suspended in complete media (with 100 μg ml −1 streptomycin and without β-mercaptoethanol). Peripheral blood-derived mononuclear cells were activated for 2 days with anti-human CD3 Ab (2 μg ml −1 ; catalogue number 16-0037-81, OKT3; eBiosciences) and anti-CD28 Ab, then expanded for 5 days with recombinant human IL-2 (300 IU ml −1 ; Novartis). All Ab and cytokines were azide and endotoxin-free. DC vaccination was performed to activate CD8 + CD44 + T cells in vivo . Mouse bone marrow-derived DCs were generated by culturing bone marrow cells for 8 days in media used for murine T-cell activation, supplemented with murine granulocyte–macrophage colony-stimulating factor ( ∼ 20 ng ml −1 ; provided by Dr Kelvin Lee, Roswell Park Cancer Institute). DCs were matured by LPS treatment (0.5 μg ml −1 ) overnight, then pulsed with 5 μM SIINFEKL peptide (InvivoGen) and 3 × 10 6 DCs were injected into the hind footpad; T cells were recovered from draining nodes (popliteal and inguinal) after 7 days. As an alternative method for in vivo activation, T cells were analysed in draining nodes (inguinal) 7 days after B16-OVA tumour implantation. Treatment with STT and LPS or neutralizing reagents Mice were treated with systemic thermal therapy (STT; core temperature of 39.5±0.5 °C, 6 h) and allowed to return to baseline temperature before homing studies as described [14] , [27] . LPS (1 mg kg −1 ; Sigma) was injected intraperitoneally (i.p.) 6 h before trafficking studies [14] . Neutralizing polyclonal anti-CXCL9 or anti-CXCL10 Ab [30] (100 μg per mouse) or polyclonal isotype IgG control (catalogue number BE0091, 100 μg per mouse; BioXCell) were injected i.p. 3 h before competitive homing studies. Murine activated CD8 + T cells were pretreated with PTX (100 ng ml −1 , 2.5 h; Sigma), or anti-mouse CXCR3-blocking Ab (catalogue number 126526, 100 μg ml −1 , 1 h; Biolegend). Human activated T cells were pretreated with PTX, human CXCR3 functional-blocking Ab (catalogue number LS-C6283-500, 40 μg ml −1 , 30 min; LifeSpan BioSciences, Inc. [39] ) or human recombinant CXCL10 (500 nM, 30 m; Peprotech), to desensitize CXCR3 (ref. 40 ). Quantification of tissue and intravascular chemokines Soluble extracts from tumour or normal skin were prepared by dissociating tissue by Medimachine (BD Biosciences) in the presence of protease inhibitors (CalBiochem). Chemokines were measured by ELISA (R&D Systems and Antigenix) or Luminex (Procarta) and normalized to total protein concentrations determined by Bradford analysis (Bio-Rad) [14] . Normal skin samples were from mice that received a s.c. injection of 100 μl sterile PBS 12 day before tissue harvest, to mimic any needle-derived inflammation at the injection site. Intravascular chemokines were detected by adapting methodology used to identify intravascular adhesion molecules in the lymph node [28] . Briefly, yellow–green fluorescent sulfate microspheres (Ex/Em 505/515, 1.0 μm diameter, Life Technologies) were labelled with 10 μg ml −1 of Ab specific for mouse chemokines including anti-CXCL10 (catalogue number MAB466-500, clone 134013), anti-CXCL9 (catalogue number AF392, affinity-purified polyclonal Ab), anti-CCL5 (catalogue number MAB478, clone 53405), anti-CCL2 (catalogue number BAF479, biotinylated affinity-purified polyclonal goat Ab) or isotype-matched control Abs (R&D Systems) and injected i.v. into tumour-bearing mice. After 1 h, tumour and pancreas were frozen in optimum cutting temperature compound (Sakura Finetek) and then counterstained using anti-mouse CD31 Ab (catalogue number 550274, clone MEC 13.3, 20 μg ml −1 ; BD Biosciences) followed by an Aminomethylcoumarin fluorochrome-conjugated goat anti-rat secondary Ab (catalogue number 112-155-003, 1:50; Jackson ImmunoResearch). For consistency, fields containing a minimum of one fluorescent bead were imaged by observers blinded to sample identity and the number of fluorescently beads associated with CD31 + vessels was quantified in ≥10 fields (unit area per field, 0.34 mm 2 ) using Image J software ( http://rsb.info.nih.gov/ij ) as described [14] . Flow cytometry Multiparameter flow cytometric analysis of murine immune cell phenotype was performed by staining with the following monoclonal Ab: anti-CD44 (catalogue number 561859, clone IM7, fluorescein isothiocyanate (FITC), 1:50), anti-CD11a (catalogue number 553120/558191, clone 2D7, FITC/phycoerythrin (PE), 1:100), anti-CD8a (catalogue number 553036, clone 53-6.7, PerCP, 1:100; catalogue number 552877, clone 53-6.7, Pe-Cy7, 1:500), anti-CD11b (catalogue number 561098, clone 1M/70, PE-Cy7 1:100), anti-Ly6C (catalogue number 560595, clone AL-21, APC, 1:100), anti-CCR5 (catalogue number 559923, clone C34-3448, PE, 1:20), anti-CD45.1 (catalogue number 560578 clone A20, PE-Cy7, 1:100), anti-CD45.2 (catalogue number 560695, clone 104, PE, 1:100) and CD3 (catalogue number 555274, clone 17A2, FITC, 1:100) (BD Biosciences); anti-CXCR3 (catalogue number FAB1685A, clone 220803, APC, 1:5), anti-CCR2 (catalogue number FAB5538A, clone 475301, 1:5) (R&D Systems); anti-granzyme B (catalogue number 50-8898, eFluor660, 1:100), anti-IFN-γ (catalogue number 17-7311-82, clone XMG1.2, APC, 1:100) (eBioscience); and anti-CD115 (catalogue number 130-102-554, clone AFS98, PE, 1:20) (Miltenyi). Functional P-selectin and E-selectin ligands were detected with CD62P or CD62E-IgG fusion proteins, respectively (catalogue number 737-PS/575-ES, 1:50, R&D Systems). Human T cells were stained with the following Ab: Zombie UV Fixable Viability Kit (Biolegend); anti-CD4 (catalogue number 563550, clone SK3, BUV395, 1:25), anti-CD3 (catalogue number 552851, clone SP34-2, PerCP, 1:20), anti-CD8 (catalogue number 557945, clone RPA-T8, Alexa Fluor 700, 1:20), anti-CCR7 (catalogue number 557648, clone 3D12, PE-Cy7, 1:20), anti-CD28 (catalogue number 563075, clone CD28.2, BV510, 1:20), anti-CD45RA (catalogue number 562885, clone HI100, BV421, 1:20) (BD Biosciences); anti-CCR2 (catalogue number 558406, clone 48607, Alexa Fluor 647, 1:5), anti-CCR5 (catalogue number 556042, PE, 1:5) and anti-CXCR3 (catalogue number 50967, APC, 1:5) (R&D Systems). Flow cytometric analysis was performed on BD LSR2 flow cytometer (BD Biosciences); compensation and analysis were performed using Winlist 6.0 (Verity Software House, Inc.). Chemotaxis assays Chemotaxis of murine and human effector T cells was assayed in 24-well plates (5 μM pore size transwell insert with polycarbonate membranes; Corning). Media alone (RPMI 1640+1% BSA) or media containing recombinant chemokines (Peprotech) was placed at the bottom of triplicate wells. Murine T-cell migration was assessed at 10 nM murine CXCL10, 1 nM murine CCL2 and 10 nM murine CCL5; human T-cell chemotaxis was determined at 100 ng ml −1 recombinant human or murine chemokine [20] unless otherwise indicated. Cells (5 × 10 5 ) were fluorescently labelled with 5- (and 6)- carboxyfluorescein diacetate succinimidyl ester (CFSE) or cell tracker orange (CTO), placed on the transwell insert and incubated at 37 °C for 3 h. Cells in the bottom chamber were enumerated by flow cytometry using Flow Count Beads (Beckman Coulter). Spontaneous migration was subtracted from all conditions and data were reported either as absolute number of cells migrated or as migration relative to WT T cells. In vivo homing assays Competitive short-term (1 h) homing assays were performed by co-mixing (1:1 ratio) 2.5 × 10 7 murine CD8 + T cells labelled with CFSE, with equal numbers of murine CD8 + T cells labelled with 5- (and 6)- (4-chloromethyl) benzoyl) amino) tetramethylrhodamine (CellTracker Orange, Invitrogen Life Technologies) before i.v. adoptive transfer. In homing studies using ex vivo activated human T cells, ∼ 1.5 × 10 7 of CFSE- or CTO-labelled cells were mixed at equivalent numbers before injection into tumour-bearing mice. Tumour and spleen were collected 1 h later and mechanically dissociated by Medimachine (BD Biosciences) or passed through a 70-μm nylon cell strainer (BD Biosciences). Ratios of fluorescent adoptively transferred cells were determined by flow cytometry and total cell numbers were assessed using Flow Count Beads (Beckman Coulter) [14] . In selected experiments, intratumoral infiltration by OT-I cells was monitored using tracking dyes (CellVue Claret, Sigma Aldrich) or by congenic mismatch (CD45.1 + OT-I→CD45.2 + host) up to 3 weeks after transfer. Quantification of extravasation by transferred CD8 + T cells After short-term in vivo homing assays, organs were harvested, embedded in optimum cutting temperature compound (Sakura Finetek) and snap-frozen as previously described [14] . Tissue cryosections (9 μm) were incubated with the primary Ab specific for murine CD31 (catalogue number 550274, clone MEC 13.3, 20 μg ml −1 ; BD Biosciences) followed by an aminomethylcoumarin fluorochrome-conjugated goat anti-rat secondary Ab (catalogue number 112-155-003, 1:50; Jackson ImmunoResearch) and imaged using a fluorescence microscope (Olympus Optical) and a SPOT RT camera (Diagnostic Instruments). In experiments in which the location of homed cells was determined (that is, extravasated versus vessel associated), all T cells not in contact with CD31 + endothelial cells were designated as extravasated. For consistency, fields containing a minimum of one fluorescently labelled cell were imaged by observers blinded to sample identity and labelled cells were quantified in ≥10 fields (unit area per field, 0.34 mm 2 ). Inflammatory monocyte isolation and short-term homing Tibias and femurs from either WT C57BL/6 or Ccr2 −/− mice were removed sterilely and the bone marrow was flushed with sterile PBS. Red blood cells were lysed with ACK lysing buffer (Gibco) and inflammatory monocytes were isolated on an AutoMacs machine using positive selection with CD115 microbeads (Miltenyi). WT CD115 + cells were labelled with CTO and Ccr2 −/− CD115 + cells were labelled with CFSE, mixed at a 1:1 ratio, and adoptively transferred into B16-OVA-bearing mice. After 2 h, tumour and splenic tissues were analysed for flow cytometry. Intravital microscopy Live imaging of tumour or normal tissues was performed as described [14] , [27] . Briefly, dorsal skin-flap single-sided window chambers (Research Instruments, Inc.) were surgically implanted in C57BL/6 mice and 1 × 10 5 B16-OVA cells were injected into the centre of the chamber. Mice were housed in a 30 °C environmental chamber, to promote wound-healing, and the adhesive qualities of the tumour microvasculature was evaluated ∼ 14–21 days post implantation. In the indicated studies, T-cell interactions were also examined in non-tumour inflamed skin vessels. Following treatment of the mice with STT or LPS, mice were anaesthetized (1 mg ml −1 xylazine and 10 mg ml −1 ketamine; 10 ml kg −1 , i.p.) and 5–10 × 10 7 calcein-labelled effector WT or Cxcr3 −/− OT-I T cells were injected via tail vein over the 30-min observation period. An epi-illumination intravital microscope with a custom stage equipped with a warming pad and vibration dampening system (Spectra Services) was used to visualize the interactions between the circulating T cells and the microvasculature. Images were captured with an EB charge-coupled device camera (Hamamatsu Photonics) and recorded with a digital videocassette recorder (DSR-11; Sony) and quantified by observers blinded to treatment conditions. T-cell interactions were quantified in unbranched vascular segments 100 μm in length with a diameter between 5 and 40 μm. The rolling fraction was the percentage of total cells that interacted per microvessel; sticking fraction was the percentage of rolling cells that subsequently adhered for ≥30 s −1 (refs 14 , 27 ). In vitro and in vivo cytotoxicity assays OVA-expressing target cells (either splenocytes pulsed with 5 μg ml −1 SIINFEKL peptide (InvivoGen), B16-OVA cells or EG7 cells) were labelled with CFSE and mixed at a 1:1 ratio with CTO-labelled non-antigen-expressing cells (that is, non-pulsed splenocytes, B16 cells or EL4 cells, respectively) and incubated in triplicate in the absence of effector T cells, or in the presence of a 15-fold excess of effector WT OT-I or Cxcr3 −/− OT-I T cells. After 24 h, live cells were analysed by flow cytometry. For in vivo cytotoxicity assays, OVA-pulsed and non-pulsed splenocytes were mixed at a 1:1 ratio ( ∼ 4–5 × 10 6 of each population per mouse) and transferred i.v. into naive mice in which 3 × 10 7 WT or Cxcr3 −/− effector OT-I T cells had been injected 3 h previously. Twenty-four hours later, spleens were harvested, lysed and live cells were analysed by flow cytometry. The proportion of fluorescently labelled cells was plotted as CFSE + and CFSE − cells on histograms, and the % specific cytotoxicity was determined by the formula (1−(% CFSE − cells/% CFSE + cells)) × 100%. Tumour growth studies WT or Cxcr3 −/− OT-I effector T cells (5 × 10 6 per mouse) were transferred i.v. into B16-OVA-bearing mice. Experimental endpoints were reached when tumours exceeded 20 mm diameter or mice became moribund. Tumour volumes were calculated by determining the length of short ( l ) and long ( L ) diameters (volume= l 2 × L /2) as described [14] . Statistical analysis All data shown are the mean±s.e.m. and group differences were evaluated by unpaired two-tailed Student’s t -test as described, unless otherwise specified. Statistical significance of tumour growth was determined by two-way analysis of variance for repeated measures. Survival data were analysed using Kaplan–Meier log rank tests. P -values <0.05 were considered significant. How to cite this article: Mikucki, M. E. et al . Non-redundant requirement for CXCR3 signalling during tumoricidal T-cell trafficking across tumour vascular checkpoints. Nat. Commun. 6:7458 doi: 10.1038/ncomms8458 (2015).